Fossil pollen records reveal a late rise of open-habitat ecosystems in Patagonia The timing of major turnovers in terrestrial ecosystems of the Cenozoic Era has been largely interpreted from the analysis of the assumed feeding preference of extinct mammals. For example, the expansion of open-habitat ecosystems (grasslands or savannas) is inferred to have occurred earlier in Patagonia than elsewhere because of the early advent of high-crowned teeth (hypsodont) mammals ∼ 26 Ma ago. However, the plant fossil record from Patagonia implies another evolutionary scenario. Here we show that the dominance of key open-habitat species—amaranths, Ephedra , asters and grasses—occurred during the last 10 Ma, about 15 Ma later than previously inferred using feeding/habitat ecology of extinct mammals. This late rise of open-landscapes in southern South America brings into question whether the expansion of open-habitat vegetation could have been the prime factor of high-crowned mammal diversification. Southern South America has yielded one of the most diverse mammalian faunas of the Neogene [1] , yet the vegetational context of their evolution has remained conjectural because of the lack of direct data. There is a widespread belief that the precocious advent—about 26 Ma ago—of fossil hypsodont mammal taxa presumed to have been feeding on grass is reflecting the earlier expansion of grasslands in southern South America than elsewhere [2] , [3] , [4] , [5] , [6] . In this study, the discovery of fossil pollen assemblages preserved in shallow marine palaeoenvironments in eastern Patagonia allowed us to explore more directly the vegetation context during the earliest dominance of hypsodont mammals. We sampled nine well-constrained stratigraphic sections exposed at Chubut and Santa Cruz provinces that span the past 26 Ma ( Supplementary Fig. S1 ). Each sample was scored for the frequency of the six ecologically most important taxa (that is, Podocarpaceae (podocarps), Nothofagaceae (southern beeches), Amaranthaceae (amaranths), Ephedraceae ( Ephedra ), asters (Asteraceae), and grasses (Poaceae)) that occur today in Patagonia, and appear to have done so throughout much of the Cenozoic [7] . We arranged pollen data in a 80-sample by 6-taxon matrix in which each cell contained the proportions of selected taxa at a sample. We applied a number of multivariate techniques (R- and Q-mode cluster analysis, non-metric multidimensional analysis or non-metric multidimensional scaling (NMDS), and a simultaneous correlation analysis of the selected species) with the aim of obtaining a better picture of what vegetation looked like during the last 26 Ma. Our analysis reveals that humid-demanding forest species (podocarps and southern beeches) dominated the Patagonian landscapes until the mid-late Miocene, and an open-landscape dominated by arid-adapted shrubs (amaranths and Ephedra ) became dominant by the late Miocene (10 Ma). We also demonstrate that grasses were uncommon during virtually all Cenozoic times in southern South America, and that their dominance occurred much later than previously inferred using the classic faunal indicators (for example, hypsodonty index). Two-mode cluster analysis The Q-mode cluster analysis recognized two major groups of samples with similar pollen composition ( Fig. 1 ). The first and most important break among the samples separates the late Oligocene–mid Miocene samples (cluster I) from all of the younger ones (cluster II). This break is also supported by a cluster analysis with significance testing ( Supplementary Fig. S2 ). The R-mode cluster leads to the recognition of two major groups of species that tend to co-occur ( Fig. 1a ); the physiognomy (namely: trees, shrubs and herbs) of the selected families, strongly affected by climatic conditions (for example, precipitation levels), appear to drive the clustering. Cluster A, linked at relatively high levels of similarity, is composed of podocarps and southern beeches (forest trees). These wet-dependent groups grow today in Patagonia along a narrow strip in the Andes where rainfall is sufficient ( ∼ 2,000 MAP) to support these and other rainforest taxa [8] . Cluster B, in contrast, is composed of asters, amaranths, Ephedra and grasses, most of them distributed in treeless habitats (steppe group). For example, Ephedra and amaranths, linked at high similarity in cluster II, occupied semi-arid to arid regions, tolerating harsh condition of <200 mm of rainfall annually [9] . With the Q- and R-mode cluster data arrayed as axes on the two-mode clustering, a pronounced floristic transition from the interval 26–16 Ma (late Oligocene–mid Miocene) to 10 Ma–18 Ka (late Miocene–Quaternary) is revealed ( Fig. 1 ). The flora of the cluster A (forest taxa) is concentrated in cluster I (late Oligocene–mid Miocene), while the flora of cluster B (steppe-taxa) is concentrated in cluster II (late Miocene–Quaternary). It thus seems clear that the abundance of canopy taxa, reflecting humid conditions and closed habitats, diminishes upwards and becomes replaced by steppe-taxa (especially Ephedra and amaranths), reflecting more arid conditions and open habitats. This replacement occurs close to the mid-late Miocene boundary. Grasses were apparently not abundant before the late Quaternary in the southernmost latitudes of South America. 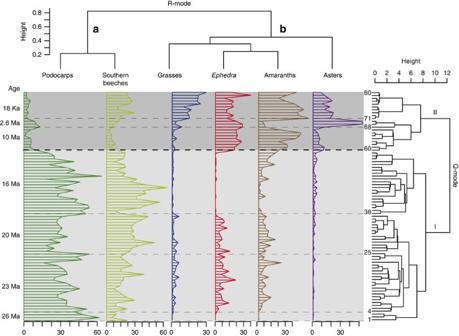Figure 1: Two-mode cluster dendrogram plot of samples and taxa derived from Bray–Curtis dissimilarity indices. The Q-mode cluster of samples—constrained by stratigraphic order—recognizes two main groups of samples from 1 to 59 and from 60 to 80 (26–16 and 10–0 Ma, respectively). Dashed-lines represent a gap of time between the adjacent sampling units. Age-constraints are given inSupplementary Table S1. The R-mode cluster recognizes two well-defined groups of physiognomic types: the wet-demanding group (a) containing rainforest trees (podocarps and southern beeches) and the arid-adapted group (b) containing steppe elements (grasses,Ephedra, amaranths and asters). The analysis of the two-mode cluster shows an important interruption in the structure of the vegetation from one dominated by rainforest species (I) to one dominated by open-habitat species (II). Even though grasses were uncommon throughout the interval selected, the remaining steppe elements were abundant during the interval 23–20 Ma (samples 4 to 37) and dominant during the interval 10–0 Ma (samples 60 to 80). Figure 1: Two-mode cluster dendrogram plot of samples and taxa derived from Bray–Curtis dissimilarity indices. The Q-mode cluster of samples—constrained by stratigraphic order—recognizes two main groups of samples from 1 to 59 and from 60 to 80 (26–16 and 10–0 Ma, respectively). Dashed-lines represent a gap of time between the adjacent sampling units. Age-constraints are given in Supplementary Table S1 . The R-mode cluster recognizes two well-defined groups of physiognomic types: the wet-demanding group ( a ) containing rainforest trees (podocarps and southern beeches) and the arid-adapted group ( b ) containing steppe elements (grasses, Ephedra , amaranths and asters). The analysis of the two-mode cluster shows an important interruption in the structure of the vegetation from one dominated by rainforest species (I) to one dominated by open-habitat species (II). Even though grasses were uncommon throughout the interval selected, the remaining steppe elements were abundant during the interval 23–20 Ma (samples 4 to 37) and dominant during the interval 10–0 Ma (samples 60 to 80). Full size image Non-metric multidimensional scaling The distances among samples in ordination space ( Fig. 2 ) further support dissimilarities between clusters I and II. Samples representing the interval 26–16 Ma (late Oligocene–mid Miocene) plot far to the right on the NMDS axis 1 because of their dominance of the wet-dependent southern beech and podocarp trees. In contrast, samples representing the interval 10 Ma–18 Ka (late Miocene–Quaternary) plot far to the left on the NMDS axis 1 due to their dominance of steppe-adapted taxa. Interestingly, asters, Ephedra , amaranths and grasses all have similar scores on axis 1, implying probable similar habitat preferences (that is, open habitats). 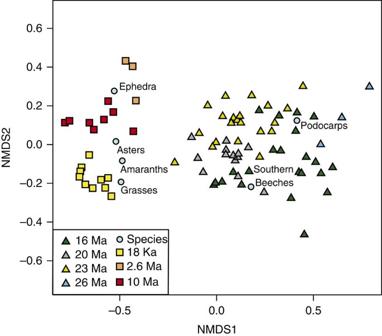Figure 2: Non-metric multidimensional scaling (NMDS) plots of each sample separately. These samples are contained in seven sampling units significantly different from each other (Analysis of Similarity R: 0.7419,P<0.001). Note that samples from 26 to 16 Ma (closer to forest species) and 10 Ma–18 Ka (closer to open-habitat species) are well separated in ordination space, with no overlapping. Scores for taxa are plotted on the same axes to better visualize the ordination in space between species and samples. Figure 2: Non-metric multidimensional scaling (NMDS) plots of each sample separately. These samples are contained in seven sampling units significantly different from each other (Analysis of Similarity R: 0.7419, P <0.001). Note that samples from 26 to 16 Ma (closer to forest species) and 10 Ma–18 Ka (closer to open-habitat species) are well separated in ordination space, with no overlapping. Scores for taxa are plotted on the same axes to better visualize the ordination in space between species and samples. Full size image Bivariate correlation analysis The correlation analysis ( Supplementary Fig. S3 ) reveals, as expected, a statistically strong positive correlation among virtually all members of the arid group. The weak correlation among species of the humid group (podocarps and southern beeches) may be related to different climatic adaptations. For example, podocarps only survive under very humid conditions, while southern beeches may tolerate seasonally dry conditions [8] . The strongest inverse correlation scores are found between Ephedra and podocarps, and between amaranths and podocarps, probably reflecting ecological extremes. The variations in the relative frequencies between forest and steppe species through time are plotted to better visualize major vegetation turnovers ( Fig. 3 ). Overall, the relative distribution of forest and steppe-taxa is relatively constant throughout much of the earlier time interval (Oligocene to early Miocene), and this distribution then becomes inverted in the time interval from the late Miocene until the present day. 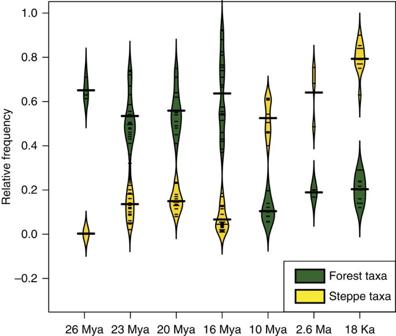Figure 3: Bean-plots showing the difference in distribution of steppe and forest species for different sampling units. A per-bean average is drawn. Note the inversion in the distribution of forest and steppe species by 10 Ma. Figure 3: Bean-plots showing the difference in distribution of steppe and forest species for different sampling units. A per-bean average is drawn. Note the inversion in the distribution of forest and steppe species by 10 Ma. Full size image The unique and detailed record of fossil pollen from Patagonia reveals a significant interruption in the structure of the vegetation from one dominated by rainforest species (late Oligocene–mid Miocene) to one dominated by open-habitat species (late Miocene–Quaternary). Our results further demonstrate that grasslands were absent in the Patagonia before the Quaternary, and that a virtually grassless ground cover of Ephedra , amaranths and asters were dominant following the local disappearance of forests by the late Miocene. The explosive radiation of hypsodont mammals (usually presumed to have been fed on grass) in a virtually grassless and canopy-dominated Patagonian environment is intriguing. Patches of open vegetation did occur within the forested matrix since (at least) the Oligocene; for example, wetland communities dominated by sedges (that is, Cyperaceae) and bulrushes (that is, Typhaceae) may have formed large and open areas within the tree-dominated landscape. This is supported by high pollen percentages of these families, reaching local dominance in some inland regions from Patagonia [7] , [10] . Furthermore, the consistent presence of amaranths and Ephedra before the local extinction of forest, in particular during the interval 23–20 Ma ( Fig. 1 ) supports the presence of a low-stature vegetation in salt-stress and alkali-stress areas (for example, coastal salt-marshes and probably some inland pockets). Nonetheless, our data indicate that Patagonia was dominated by forest taxa by the late Oligocene–mid Miocene interval on the basis of the fossil pollen record ( Fig. 4 ). 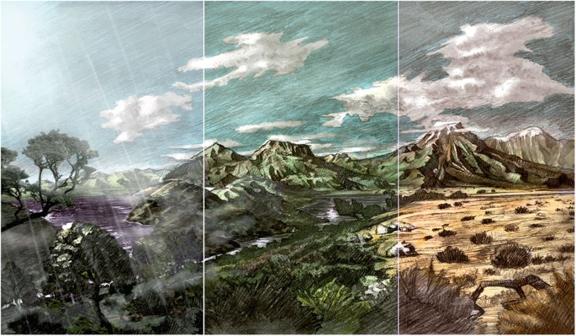Figure 4: Patagonian landscapes through different periods. Reconstruction of successive Patagonian landscapes during the last 26 Ma, from the humid and tree-dominated late-Oligocene (left) to the arid and treeless present-day (right). Figure 4: Patagonian landscapes through different periods. Reconstruction of successive Patagonian landscapes during the last 26 Ma, from the humid and tree-dominated late-Oligocene (left) to the arid and treeless present-day (right). Full size image The scarcity of fossil grass pollen in the Patagonian pre-Pliocene record compared, for example, to aster pollen, also dominant in present-day open habitats, implies either: (1) grass pollen is rarely preserved; (2) grass pollen is frequently overlooked/misidentified; or (3) grass pollen was scarce in these ecosystems. Hypotheses 1 and 2 can be rejected because grass fossil pollen is recorded since, at least, the Palaeocene, and because it can be unambiguously assigned at the family level [11] . Hypothesis 3 seems the most convincing; before grasses became ecologically dominant, shrubs and herbs of asters, amaranths and Ephedra might have had the pioneering role in repopulating the vast and deforested late Miocene Patagonian landscapes. Although, these shrubs, particularly Ephedra , became confined to the driest regions of the present-day Patagonian desert, other minor components that also formed part of the sclerophyllous communities of the late Miocene, did not survive. For example, some members of the Vivianiaceae (for example, Viviania marifolia and Viviania albiflora ) and the aster family (for example, Schlechtendalia luzulaefolia , and Holocheilus – Proustia – Jungia group) became locally extinct probably in response to the subsequent climatic deterioration (that is, glacial periods of the Quaternary). For this reason, during the last 10 million years the southern range limit of these taxa contracted northward (northeastern Argentina, Uruguay and Brazil) and/or westward (western Argentina and Chile), probably retaining their ecological preferences [12] , [13] , [14] , [15] (Niche Conservatism?). Overall, these data suggest a late Miocene open-landscape, probably warmer than today at the same latitude. As mentioned earlier, sedges and bulrushes were also frequent during these times, indicating the presence of humid spots (for example, ponds or permanently saturated soils), where some locally extinct mammals lived, including the Hydrochoeridae (for example, capybaras) [16] . Apart from fossil pollen records, several recent lines of data point towards a woody rather than a grassy landscape during the late Oligocene–Miocene interval, such as the local distribution of fossil phytoliths preserved in sediments. Phytoliths are particles of hydrated silica formed in living plants that are liberated after they die and decay [17] . Unlike pollen remains, phytoliths are incorporated into the soil through the decay of leaf litter, providing very specific local information. The fossil record of phytoliths from the Patagonian fossiliferous site ‘Gran Barranca’ (central Patagonia), where the most complete sequence of middle Cenozoic palaeo-faunas in South America is exposed [18] , has been the subject of some debate during the last years. Former studies suggested grass-dominated ecosystems during mid Eocene, including the presence of C 4 grass lineages [19] . Later analysis, however, seems to favour the assumption that palms and woody dicotyledons dominated phytolith assemblages at the ‘Gran Barranca’ site during the Eocene-early Miocene [20] . Moreover, the lack of C 4 grasses in Patagonia was previously pointed out by MacFadden et al . [21] who analysed the tooth enamel of extinct herbivores and concluded that high-crowned hypsodonts from southern South America occurred under a regime of C 3 photosynthesis. All these data, along with the fact that frugivores, insectivores and omnivores, including platyrrhine primates were common during the Miocene of Patagonia, indicate that forests persisted across Patagonian landscapes. Regional and global forcing may have had a role in triggering these floristic shifts, by eliminating more than 500,000 km 2 of forests and giving rise to the Americas’ most widespread desert. In this scenario, the Andean uplift is inferred as having acted as the major driving mechanism by blocking the passage of rain-producing systems from the west, casting a shadow of dryness on the lee side of the Andes since at least the late Miocene. Global cooling events are also known to have triggered significant shifts in aridity during the Cenozoic [22] . In this context, the two major expansions of ice-sheets on Antarctica [23] mirror the increase of open-habitat species in Patagonia during the earliest Miocene (23–20 Ma) and more significantly since the late Miocene (10 Ma). Whether the Andean uplift or the global drop in temperatures represents the prime driver of aridity in southern South America remains to be tested. It seems reasonable to assume that the Andean uplift reduced seasonal precipitation on the leeward side of the mountains, while low global sea levels, corresponding to glacial Antarctic events of the Miocene, enhanced the increased continental aridity. The timing of the onset of aridification inferred from the Patagonian fossil pollen record fully agrees with that from Australia [24] , Africa [25] , North America [26] , Europe [27] and Asia [28] on the basis of sedimentological and/or palaeontological analyses. This points to a major establishment of the world’s most important open-habitat systems during a relatively small window of time by the late Miocene/Pliocene. Even though our picture of Patagonia contrasts markedly with the traditional beliefs of an early emergence of grasslands by the Oligocene on the basis of the advent of high-crowned hypsodont mammals, complementary approaches (for example, tooth wear scoring methods) have been giving new insights. For example, Townsend and Croft [29] using a microwear analysis assessed the feeding preferences of three species of Notoungulata from the Miocene of Patagonia, typically assumed to be grazers because of their high levels of hypsodonty. They concluded that these extinct mammals were primarily feeding on browse (that is, eating the leaves and stems of dicotyledonous plants, such as trees, shrubs or bushes) and pointed out that hypsodonty cannot tell us whether or not an animal could have been a strict grazer; rather, they stressed that palaeoecology must be assessed on a case by case basis to evaluate its role in feeding [29] . Although we are unable to challenge the adaptive value of hypsodonty from the fossil pollen analysis, we demonstrate quantitatively that grasslands per se were virtually absent prior to Quaternary in Patagonia: thus, whatever the results of the microwear analysis, these animals could not have been eating grass. Kaiser et al. [30] showed that external abrasives of very fine particle size have a major role in naturally occurring tooth wear, which is consistent with the view of Pascual and Ortiz Jaureguizar [31] , who interpreted precocious hypsodonty in South American ungulates as an effective response to abrasive volcanic ash that may had dusted the leaves of plants. The present study adds a key piece to an intriguing puzzle by incorporating a new floristic context for much of the evolutionary history of mammalian herbivores in southern South America. Future efforts will concentrate on enhance interdisciplinary collaborations between palaeobotanists and palaeozoologists to better identify and potentially correlate the most significant turnovers between floras and faunas during the Neogene. Understanding the past interactions among species during past instances of biological diversifications will enable us to recognize present and future responses to unpredicted scenarios. Sampling Detailed palynological analyses of six sampling units represented by nine sections exposed at southeastern Argentina were undertaken for reconstruction of palaeovegetation of the past 26 Ma. Fossil pollen analysis has proved to be the best suited palaeoecological approach to test hypotheses about what major vegetation belts co-occurred, either at a regional or at a more local scale. A regional-level reconstruction, in particular, may be addressed best by analysing the fossil pollen contained in coastal-marine deposits [32] . This is because coastal or marginal marine environments preserve a reasonably accurate representation of the pollen derived from adjacent lands, with little of the complicating fluctuation of local input present in terrestrial records (swamp and lake sediments). The nine sampled sections are Punta Nava (30 m), Cerro Chenque (208 m), Punta Delgada (38 m), Cerro Viteau (117 m), Playa Las Cuevas (15 m), Cerro Antena (89 m), Cañadón Baumann (64 m), Punta Pirámide (15 m) and Restinga Norte (10 m). Overall, these sections primarily consist of fine-grained sandstones, coquinas and heterolithic (fine-grained sandstone interbedded with mudstones) beds. The geological setting, stratigraphy, depositional environment and age-constraint of the sampling units have been analysed in detail elsewhere [33] , [34] , [35] , [36] and summarized in Supplementary Table S1 . We collected and processed 405 samples and performed quantitative and taxonomic palynological analyses on 165 samples from which we selected 70 to better represent the landscape-level vegetation. These selected samples contain dinoflagellate cysts as well as fluvial- (for example, Cyperaceae, Azolla, Typhaceae-Sparganiaceae), broad-regional- (for example, Nothofagaceae, Podocarpaceae, Asteraceae, Amaranthaceae, Poaceae) and restricted- (for example, Poteaceae, Fabaceae) dispersal types. For comparison purposes, we selected from the literature a late Quaternary analogue of 10 samples [37] . Standard palynological techniques were used to process all samples [38] . We counted from 250 to 300 individuals per slide. All slides and residues are housed at the palynotheca of the Museo Argentino de Ciencias Naturales ‘Bernardino Rivadavia’. Age calibration Biostratigraphic and radiometric constraints on sampling units are given in Supplementary Table S1 . Selected taxa We selected plant families common across Patagonia during much of the Cenozoic. These are the amaranth (Amaranthaceae), aster (Asteraceae), Ephedra (Ephedraceae), southern beech (Nothofagaceae), grass (Poaceae) and podocarp (Podocarpaceae) families. All these families (1) consist of wind-pollinated taxa that produce copious amounts of easily dispersed pollen grains, (2) produce morphologically distinctive pollen types and (3) today occupy ecologically defined floristic formations (that is, rainforest or steppes). The most common fossil taxa found in Patagonian deposits assigned to these families are Chenopodipollis chenopodiaceoides (Martin) Truswell (Amaranthaceae ), Tubulifloridites antipodica Cookson, T. simplis Martin , T. pleistocenicus Martin and Mutisiapollis viteauensis Barreda (Asteraceae), Equisetosporites claricristatus (Shakmundes) Barreda, E. lusaticus (Krutzsch) Barreda and E. notensis (Cookson) Romero (Ephedraceae), Nothofagidites spp. (Nothofagaceae), Graminidites spp. (Poaceae) and Podocarpidites spp., Phyllocladidites mawsonii Cookson and Lygistepollenites florinii (Cookson and Pike) Stover and Partridge (Podocarpaceae). Quantitative analyses The relative frequencies of the selected taxa were calculated from the total number of terrestrial spores and pollen grains. All multivariate analyses were conducted using open source R version 2.15.0 ( http://www.r-project.org/ ). All analyses were run on square root transformation, which partially reduces the problems associated with closed-sum percentage data [39] . We conducted a constrained cluster analysis (CCA) to explore sample associations (Q-mode) and a hierarchical cluster analysis (HCA) to explore taxonomic associations (R-mode). We used the Bray–Curtis distance to create a matrix of dissimilarity before running HCA. The agglomerative method used in HCA was the Ward. We used Chclust (package ‘rioja’), that performs a CCA of a distance matrix, with clusters constrained by sample order. The agglomeration method used in this CCA was the coniss. We also compared the CCA with a HCA with bootstrapped P -values (package ‘pvclust’), ensuring that artificial groupings would not be misinterpreted ( Supplementary Fig. S3 ). We ordinated the samples and species using NMDS regarded as the most robust unconstrained ordination method in community ecology [40] . The main objective of NMDS is to plot dissimilar objects far apart in the ordination space and similar objects close to one another (‘metaMDS’ function, package ‘vegan’). We conducted the Analysis of Similarity to test for significant differences between sampling units [41] . The statistic R will be in the interval −1 to +1; the value 0 indicates completely random grouping while the value +1 or close to +1 indicates that samples within sites are more similar to each other than to samples from different sites. The correlation analysis among variables was used to show whether and how strongly pairs of variables are related (‘panel.cor.res’ function, package ‘asbio’). Distributions of steppe and forest taxa were visualized using bean-plots (package ‘beanplot’). How to cite this article: Palazzesi, L. & Barreda, V. Fossil pollen records reveal a late rise of open-habitat ecosystems in Patagonia. Nat. Commun . 3:1294 doi: 10.1038/ncomms2299 (2012).